In vitrotransport activity of the fully assembled MexAB-OprM efflux pump fromPseudomonas aeruginosa Antibiotic resistance is a major public health issue and many bacteria responsible for human infections have now developed a variety of antibiotic resistance mechanisms. For instance, Pseudomonas aeruginosa , a disease-causing Gram-negative bacteria, is now resistant to almost every class of antibiotics. Much of this resistance is attributable to multidrug efflux pumps, which are tripartite membrane protein complexes that span both membranes and actively expel antibiotics. Here we report an in vitro procedure to monitor transport by the tripartite MexAB-OprM pump. By combining proteoliposomes containing the MexAB and OprM portions of the complex, we are able to assay energy-dependent substrate translocation in a system that mimics the dual-membrane architecture of Gram-negative bacteria. This assay facilitates the study of pump transport dynamics and could be used to screen pump inhibitors with potential clinical use in restoring therapeutic activity of old antibiotics. P seudomonas aeruginosa is a multi-resistant Gram-negative bacteria that is responsible for 10% of nosocomial infections [1] . Efflux pumps play a major role in the development of multidrug resistance by actively exporting a wide variety of noxious compounds outside of the bacteria. In 2000, sequencing of the genome of P. aeruginosa led to the identification of at least 12 efflux pumps [2] . The constitutively expressed tripartite efflux pump consists of the following: MexB, a protein from the resistance-nodulation-division family (RND) located within the inner membrane that binds the antibiotic and initiates its transport using the proton motive force [3] ; MexA, a membrane fusion protein (MFP), attached to the inner membrane with a lipid anchor, found in the periplasmic space, that is essential for in vivo transport and pump assembly [4] , [5] ; and OprM, a channel from the outer membrane factor family (OMF) located in the outer membrane that allows the extrusion of antibiotics [6] . High-resolution structures have been described for the various components [3] , [4] , [5] , [6] and shed light on the molecular determinants of transport. However, the understanding of how the pump is assembled and functions urgently requires new tools. Such tools would be very useful as it has been demonstrated that inhibition of multidrug resistance pumps increases antibiotic susceptibility [7] and reduces the probability of the emergence of antibiotic resistant mutants [8] . Studies investigating the in vitro activity of an efflux pump are scarce and all of them focus only on the RND and MFP. In 1999, Zgurskaya and Nikaido [9] achieved the first successful functional reconstitution of AcrB, and they showed that AcrB catalyses the extrusion of fluorescent phospholipids. Soon afterwards, the successful reconstitution of another RND, CzcA, was reported. CzcA is the RND of the efflux pump CzcCB 2 A, responsible for heavy-metal resistance in Ralstonia sp [10] . In 2010, Yu et al . described a high-resolution structure and the functional reconstitution of the RND CusA [11] . The efflux pump CusCBA is responsible for extruding biocidal Cu(I) and Ag(I) ions in Escherichia coli . All these assays were facilitated by the availability of titratable substrates (for example, fluorescent lipids and radiolabelled metals). The first challenge when studying efflux pumps is to find a relevant index of transport. In 2010, Venter and colleagues [12] showed that the transport of Hoechst 33342, a known substrate of efflux pumps, can be monitored. However, much care must be taken when manipulating this molecule in solution because its fluorescence and lipophilicity are highly dependent on the pH of the medium [13] . Therefore, in vitro studies on efflux pumps most often rely on a secondary reporter probe, specifically, the pH variations inside the liposome followed by the use of a pH-dependent fluorescent probe such as pyranine [9] , [14] , [15] , [16] , [17] . Lately, we have optimized a functional test where the activity of MexB was indirectly monitored by measuring the pH inside proteoliposomes in which MexB was reconstituted in the presence or in the absence of MexA [16] , [17] . Energization of the system was achieved after the vectorial incorporation of bacteriorhodopsin, a light-activated proton pump. Setting up an in vitro test for the tripartite efflux pump has long been thought to be a complicated task. We present here the design of an experimental setup to assay the entire MexA-MexB-OprM efflux pump. First, we showed that the substrate is recruited by the MexAB proteoliposome, is processed by the entire pump and reaches the lumen of the OprM proteoliposome. Then, we evaluated the mutual interplay of the three protein partners. We demonstrate that OprM must interact with MexA and MexB to open, a result that is in accordance with a previous model [6] and that the activity of MexB is reciprocally improved when the pump is assembled. Design of the tripartite assay system First, pyranine-encapsulated MexAB proteoliposomes (the palmitoylated version of MexA) and RNA-encapsulated OprM proteoliposomes are mixed and ethidium bromide, a substrate of MexB that spontaneously inserts into membranes, is added to the system. Ethidium bromide is a RNA intercalating agent, which shows increased fluorescence when intercalated into RNA ( Fig. 1 ). Note that ethidium bromide is not encapsulated in the liposomes but is added to the cuvette so that it reaches MexB from outside the liposomes, that is, from the side corresponding to the periplasm. 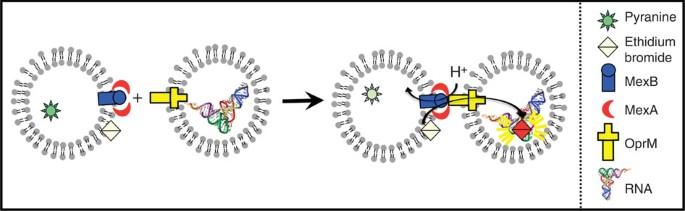Figure 1: Schematic representation of thein vitroefflux pump assembly. MexB and OprM were reconstituted in proteoliposomes and on mixing, the tripartite complex forms and transport through the whole efflux pump is monitored by the use of carefully chosen fluorescent reporters. MexA and MexB are reconstituted in proteoliposomes containing pyranine, OprM is reconstituted in another proteoliposome in which RNA is encapsulated. Ethidium bromide is a substrate of the pump that has nucleic acid-intercalating properties. Transport through the efflux pump is monitored by measuring pyranine and ethidium bromide fluorescence simultaneously. The concomitant fluorescence variations indicate actual transport of the substrate, from one vesicle to the other (increase of ethidium bromide fluorescence), mediated by an active transport through the pump (decrease of pyranine fluorescence). Figure 1: Schematic representation of the in vitro efflux pump assembly. MexB and OprM were reconstituted in proteoliposomes and on mixing, the tripartite complex forms and transport through the whole efflux pump is monitored by the use of carefully chosen fluorescent reporters. MexA and MexB are reconstituted in proteoliposomes containing pyranine, OprM is reconstituted in another proteoliposome in which RNA is encapsulated. Ethidium bromide is a substrate of the pump that has nucleic acid-intercalating properties. Transport through the efflux pump is monitored by measuring pyranine and ethidium bromide fluorescence simultaneously. The concomitant fluorescence variations indicate actual transport of the substrate, from one vesicle to the other (increase of ethidium bromide fluorescence), mediated by an active transport through the pump (decrease of pyranine fluorescence). Full size image Transport of ethidium bromide through a functional pump A proton gradient is generated, and ethidium bromide fluorescence is monitored. An increase of fluorescence is observed in liposomes in which wild-type MexAB is reconstituted ( Fig. 2 ; red trace). The increase of fluorescence demonstrates that the whole pump is assembled in vitro and that ethidium bromide is transported from one liposome to the other, via the efflux pump. As a control, MexA is reconstituted with a non-functional mutant of MexB (MexB D407N, a mutant in which proton counter-transport is compromised) to ensure that the ethidium bromide efflux is due to the action of the tripartite efflux pump by active transport via MexAB, and not by passive leakage through the membranes. Indeed, the fluorescence is steady when MexAB mutant and OprM proteoliposomes are mixed ( Fig. 2 ; blue trace). As another control, MexAB proteoliposomes are mixed with protein-free control liposomes loaded with RNA. Once again the fluorescence is steady on the generation of a proton gradient ( Fig. 2 ; black trace). As a final control, OprM RNA-loaded proteoliposomes are mixed with control liposomes and no increase of fluorescence on generation of the proton gradient is observed ( Supplementary Fig. 1 ; green trace). 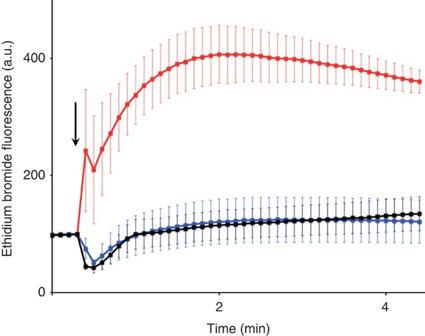Figure 2: Ethidium bromide fluorescence as a function of time. Ethidium bromide fluorescence was monitored in the liposome assay system after addition of hydrochloric acid (arrow). Red trace: wild-type MexAB and OprM proteoliposomes are mixed, blue trace: MexAB D407N and OprM proteoliposomes are mixed, black trace: wild-type MexAB and control RNA-loaded liposomes are mixed. The ethidium bromide concentration is 2 μM. Error bars represent the s.d. (n=3);λex=300 nm andλem=600 nm. Figure 2: Ethidium bromide fluorescence as a function of time. Ethidium bromide fluorescence was monitored in the liposome assay system after addition of hydrochloric acid (arrow). Red trace: wild-type MexAB and OprM proteoliposomes are mixed, blue trace: MexAB D407N and OprM proteoliposomes are mixed, black trace: wild-type MexAB and control RNA-loaded liposomes are mixed. The ethidium bromide concentration is 2 μM. Error bars represent the s.d. ( n =3); λ ex =300 nm and λ em =600 nm. Full size image In addition, we verified that proteoliposomes containing OprM are not leaky ( Supplementary Fig. 2 ; Supplementary Note 1 ). Altogether, the above experiments indicate that OprM is in a closed state on its own, which is in agreement with crystal structure data [6] , and that it opens on interaction with MexAB. Hence, the system presented here allows the observation of substrate transport when the pump is assembled. An unexpected effect of OprM on assembly . Because the efflux pump is successfully assembled in vitro , we can therefore investigate the effect of OprM on MexAB activity. To that purpose, the same transport assay described above is run, but pyranine fluorescence is also measured. As a first step, MexAB activity is investigated. We reconstituted MexAB in liposomes and monitored the pH variations using pyranine in the presence of a substrate, meropenem ( Fig. 3 ). Once again, the substrate is not loaded in the liposome, but added to the ‘periplasmic’ side of MexB before the assay. 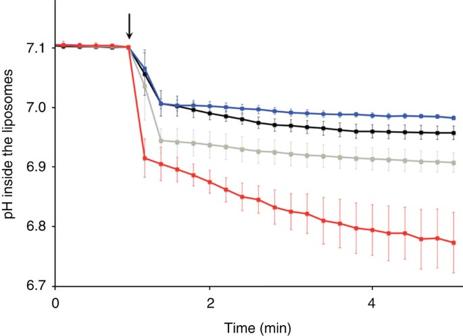Figure 3: Liposome pH as a function of time. pH inside of the liposomes was monitored in the presence of meropenem (5 μM); the arrow represents hydrochloric acid addition. Black trace: protein-free liposomes, blue trace: MexAB D407N proteoliposomes, grey trace: MexAB proteoliposomes, red trace: MexAB proteoliposomes mixed with OprM proteoliposomes. Error bars represent the s.d. (n=3). Figure 3: Liposome pH as a function of time. pH inside of the liposomes was monitored in the presence of meropenem (5 μM); the arrow represents hydrochloric acid addition. Black trace: protein-free liposomes, blue trace: MexAB D407N proteoliposomes, grey trace: MexAB proteoliposomes, red trace: MexAB proteoliposomes mixed with OprM proteoliposomes. Error bars represent the s.d. ( n =3). Full size image To be functional, MexB must be subjected to a proton gradient; in our assay, the orientation of the protein requires an acidic gradient outside of the liposome. To produce this gradient, hydrochloric acid is added outside. It is known that protons cross the lipid bilayer following biphasic kinetics in the presence of a pH gradient. A first very rapid phase corresponds to the entry of protons down the concentration gradient ( Supplementary Fig. 3a ; Supplementary Note 2 ). This rapid phase stops when the flux of protons is compensated by counterflux of protons driven by the membrane potential ( Supplementary Fig. 3b ). The second phase is slow and corresponds to the leakage of cations out of the liposomes, compensating for the entry of protons [18] . Therefore, all of the pH variations described below are biphasic ( Fig. 3 ). Depending on the presence of protein in the liposome, either the first and/or the second phase will be affected. For all types of liposomes, the pH reaches the same value after overnight incubation ( Supplementary Fig. 4 ). On generation of a proton gradient in the presence of meropenem, protons first rapidly and then slowly cross the membrane of protein-free liposomes ( Fig. 3 ; black trace) until the pH eventually reaches an equilibrium value (pH=5.8 after overnight incubation; Supplementary Fig. 4 ). However, the entrance of protons to the proteoliposomes during the first rapid phase is greatly accelerated when MexAB is reconstituted ( Fig. 3 ; grey trace). Note that the same results are obtained when ethidium bromide is used as a substrate ( Supplementary Fig. 5 ; Supplementary Note 3 ). To ensure that this more rapid acidification really is due to the transport of protons via MexAB and not to the passive leakage of protons through the protein, we have reconstituted MexA with MexB D407N. On generation of a proton gradient, it is shown that this non-functional protein leads to a signal comparable to that observed for the protein-free liposomes ( Fig. 3 ; blue trace versus black trace). Note that MexAB does not transport imipenem in vitro ( Supplementary Fig. 5 ). This observation provides additional evidence that the assay is specific because it is known that imipenem is not a substrate of MexB in vivo [19] . MFP interaction with the RND has been already investigated with both AcrAB [9] and MexAB [16] , but experimental evidence for a putative role of the OMF in transport is lacking. In this study, the effect of OprM on MexAB activity is investigated. As seen in Fig. 3 , OprM has a major effect on the activity of MexAB because the pH inside of MexAB proteoliposomes drops much faster in the presence (red trace) than in the absence of OprM (grey trace). Interestingly, in this case, both the rapid and slow phases are affected by the presence of OprM. Indeed, the pH now reaches a steady state only after ∼ 2 min. As mentioned above, after overnight incubation of all samples, the pH reaches an equilibrium value of pH=5.8 ( Supplementary Fig. 4 ). If the in vitro assay is performed without MexA, no enhancement of the activity of MexB occurs on OprM addition ( Supplementary Fig. 6 ; Supplementary Note 4 ). Finally, we also show that the effect is indeed substrate-dependent ( Supplementary Fig. 7 ; Supplementary Fig. 8 ; Supplementary Note 5 ; Supplementary Note 6 ). We can conclude that MexA could play two roles that are not mutually exclusive, corresponding to the two models of the assembly of the tripartite efflux pump presented in Fig. 4 : (i) MexA could allow the docking of MexB on OprM (OMF-RND docking model, Fig. 4a [5] ) or (ii) MexA could create a funnel link between OprM and MexB (MFP-mediated model, Fig. 4c [20] ). 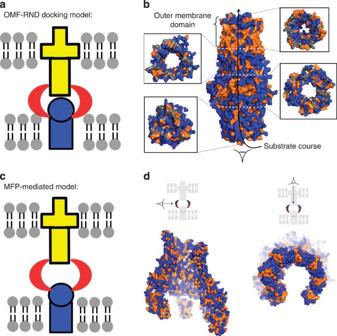Figure 4: The two main models of the efflux pump assembly. (a) OMF-RND docking model describing one of the two favoured architectures of the assembly where the RND protein, represented in blue, is in direct contact with the OMF, represented in yellow. (b) Hydrophilic (blue) and hydrophobic (orange) residues of OprM are shown as a surface representation. For a better understanding, OprM has been divided in four parts. (c) MFP-mediated model describing an alternative architecture described in the literature. In this model, the MFP protein, represented in red, makes a physical link between the RND protein, represented in blue, and the OMF, represented in yellow. (d). Hydrophilic (blue) and hydrophobic (orange) residues of the funnel-like hexamer of MexA are shown as a surface representation (right). This figure was made with Pymol. PDB accession codes: MexA1T5Eand OprM3D5K. Figure 4: The two main models of the efflux pump assembly. ( a ) OMF-RND docking model describing one of the two favoured architectures of the assembly where the RND protein, represented in blue, is in direct contact with the OMF, represented in yellow. ( b ) Hydrophilic (blue) and hydrophobic (orange) residues of OprM are shown as a surface representation. For a better understanding, OprM has been divided in four parts. ( c ) MFP-mediated model describing an alternative architecture described in the literature. In this model, the MFP protein, represented in red, makes a physical link between the RND protein, represented in blue, and the OMF, represented in yellow. ( d ). Hydrophilic (blue) and hydrophobic (orange) residues of the funnel-like hexamer of MexA are shown as a surface representation (right). This figure was made with Pymol. PDB accession codes: MexA 1T5E and OprM 3D5K . Full size image We showed that in the presence of OprM, MexB activity is enhanced and MexB pumps for a longer time, but only in the presence of MexA. This enhanced activity could be ascribed to the physico–chemical interaction of the substrate with the solvent in a confined cavity. In a recent all-atom targeted molecular dynamic simulation of AcrB [21] , it was shown that mere conformational movements of the RND (a zipper-like squeezing of the binding pocket) were not sufficient to explain the total extrusion process. This was corroborated by Imai and colleagues [22] who showed that the substrate is stabilized by a subtle free-energy balance originating in the weakly polar and weakly hydrophobic surroundings rather than by specific interactions such as hydrogen bonds. Both studies postulated that the driving force for the extrusion could be a combination of the diffusion of the substrate as well as attractive interactions between the substrate and residues within TolC. Considering that the residues lining the inner surface of TolC [23] and OprM [6] are rather polar ( Fig. 4b ), on interaction with OprM the substrate would be in an environment that might drive it out. This hypothesis is also compatible with the MFP-mediated model because MexA can provide a similar hydrophilic environment ( Fig. 4d ; left). Our data therefore are compatible with both of the models. As described above, there is a clear and unexpected effect of OprM on the kinetics of activity of MexB. This is quite counterintuitive, given that OprM actually enhances the substrate consumption. However, the effect of OprM could be explained by the structural rearrangements of MexB induced by its interaction with OprM. Indeed, once the pump is assembled, MexB might adopt a conformation that allows the recruitment of substrate at a lower concentration than in the absence of OprM. The first in vitro reconstitution of a tripartite efflux pump is presented here. This achievement is highly beneficial for the study of multidrug efflux pumps. The assay relies on the use of ethidium bromide as a substrate for MexB but this is not a limitation. Indeed, this assay could very well be adapted to any substrate because the RNA scaffold encapsulated in the OprM proteoliposomes can be modified. The RNA scaffold has a restriction site in which any nucleic acid material can be inserted [25] . Furthermore, DNA/RNA aptamers specific for an increasing number of targets are now available, and it has been shown that it is possible to rationally convert non-fluorescent aptamers into fluorescent reporters [26] . It has also been shown that fluorescent aptamers can be selected directly from random sequence DNA libraries in vitro [27] . Hence, aptamers specific for any substrate could be used as probes to monitor assembly and transport activity. Materials 1,2-Dioleoyl-sn-glycero-3-phosphocholine (DOPC), 1,2-dioleoyl- sn -glycero-3-phosphoethanolamine (DOPE) and egg L-α-phosphatidylcholine (EPC) were purchased from Avanti Polar Lipids. Cholesterol, 8-hydroxypyrene-1,3,6-trisulphonic acid (pyranine), Triton X-100 and ethidium bromide were obtained from Sigma-Aldrich. SM2 Bio-beads were obtained from Bio-Rad. n-Dodecyl-β-D-maltopyranoside and n-octyl-β-D-glucopyranoside (β-OG) were purchased from Anatrace. Protein preparation MexB is purified following the protocol described in ref. 24 with minor modifications. Heterologous expression is performed in a C43 ΔAcrB (provided by K.M Pos) strain. A pre-culture is grown overnight at 37 °C under agitation at 200 r.p.m. and inoculated at OD 600 nm =0.05 in 2 × TY medium containing 100 μg ml −1 of ampicillin. Cells are grown to OD 600 nm =0.6 at 30 °C at 200 r.p.m. and then cooled down at 4 °C for 30 min. Isopropyl β-D-1-thiogalactopyranoside is added (1 mg ml −1 final) to induce the expression of MexB. Growth is continued overnight at 20 °C. Cells are then lysed, thanks to a cell disrupter (Cell-D from Constant LTD) at 4 °C after two passages at 2.4 kbar. Membranes are collected on centrifugation at 100,000 g for 1 h at 4 °C. Solubilization is performed overnight at 4 °C in Bis-Tris 10 mM pH 7.4; glycerol 20%, imidazole 10 mM and NaCl 500 mM and at a 2:1 (w/w) detergent-to-protein ratio (protein concentration is determined using the Bicinchoninic acid test from Sigma). Purification is performed by affinity chromatography followed by a gel filtration (superose 6 HR, GE). MexA is purified following the protocol described in ref. 4 with minor modifications. Heterologous expression is performed in a C43 ΔAcrB (provided by K.M Pos) strain. A pre-culture is grown overnight at 37 °C under agitation at 200 r.p.m. and inoculated at OD 600 nm =0.05 in 2 × TY medium 25 μg ml −1 of chloramphenicol. Cell are grown to OD 600 nm =0.6 at 30 °C at 200 r.p.m. Arabinose is added (0.02% final w/w). Growth is continued for 2.5 h at 30 °C. Cells are then lysed, thanks to a cell disrupter (Cell-D from Constant LTD) at 4 °C after two passages at 2.4 kbar. Membranes are collected on centrifugation at 100,000 g for 1 h at 4 °C. Solubilization is performed overnight at room temperature in Tris-HCl 20 mM pH 8, glycerol 10%, imidazole 15 mM at a 40:1 (w/w) detergent-to-protein ratio (protein concentration is determined using the Bicinchoninic acid test from Sigma). Purification is performed by affinity chromatography followed by a gel filtration (superose 6 HR, GE). Throughout the manuscript, MexA refers to the palmitoylated version of the protein. OprM is purified following the protocol described in ref. 6 with minor modifications. In brief, the procedure is exactly that described above for MexA except that an additional solubilization step is added before membranes are collected. N-octylpolyoxyethylene (C8POE) is added (2% final) on the lysed cells and the mixture is incubated for 30 min at 37 °C. C8POE is a detergent that has been shown to specifically solubilize bacterial inner membranes. Expression and purification of the ref-f RNA scaffold were performed as described in ref. 25 with the following modifications. Heterologous expression of ref-f is achieved in XL1 cells. A pre-culture is grown 10 h at 37 °C under shaking at 200 r.p.m. and inoculated at OD 600 nm =0.05 in LB medium containing 100 μg ml −1 of ampicillin. Cells are grown overnight to OD 600 nm =3 at 37 °C at 200 r.p.m. The expression of ref-f is induced by the addition of 1 mM of isopropyl β-D-1-thiogalactopyranoside. After 3 h, cells are centrifuged at 7,000 g for 20 min at room temperature. Pellets are resuspended in 1 l of Tris 20 mM, NaCl 200 mM and centrifuged at 7,000 g for 20 min, again at room temperature. Pellets are resuspended in 40 mM of MgSO 4 10 mM, Na 3 Citrate 50 mM pH 5.6. RNA is extracted upon incubation with 40 ml of phenol for 2 h under gentle stirring at room temperature. The mixture is centrifuged for 15 min at 3,200 g . The supernatant is incubated with two volumes of ethanol and 1/20 of NaCl 5 M, a precipitate is formed and the mixture is centrifuged for 5 min at 3,200 g . The pellet is dried under the fume hood for 5 min and 10 ml of distilled water is added. The RNA is then purified by anion exchange chromatography. The solution is loaded on a Source Q column previously equilibrated with KPi 20 mM pH 6.5 and washed with 500 ml of KPi 20 mM pH 6.5, NaCl 400 mM (40% of buffer B: KPi 20 mM pH 6.5 NaCl 1 M). The RNA is then eluted, thanks to a gradient of 350 ml from 40–55% of buffer B. Preparation of unilamellar vesicules MexAB proteoliposomes are prepared as described below. Cholesterol (powder) was added to DOPC (in chloroform) and dried under vacuum. The resulting lipidic film was dissolved in HEPES 25 mM pH 7, K 2 SO 4 100 mM, MgCl 2 2 mM and pyranine 3 mM to final concentrations of 10 mg ml −1 for DOPC and 1.5 mg ml −1 for cholesterol. The suspension was heated for 10 min at 37 °C. This solution was then sonicated for 10 min. The liposomes were extruded through 200-nm membranes and through 100-nm membranes. β-OG was then added to reach a 2.5 detergent/lipid ratio (w/w). Proteins were added to the solubilized liposome suspension at the following ratios (w/w): lipids/MexB=20 and MexB/MexA=2.5. Detergent removal was achieved on addition of Bio-beads at a Bio-bead/detergent ratio of 30 (w/w). The proteoliposomes were purified using a PD-10 desalting column (GE Healthcare). The efficiency of the reconstitution should be systematically controlled by performing ultracentrifugation of the liposomes on a sucrose gradient ( Supplementary Fig. 9 ). OprM proteoliposomes are prepared as described below. DOPE and EPC in chloroform were dried under vacuum. The resulting lipidic film was dissolved in HEPES 25 mM pH 7, K 2 SO 4 100 mM, MgCl 2 2 mM and ref-f RNA 3 mg ml −1 to final concentrations of 24.4 mg ml −1 for EPC and 12 mg ml −1 for DOPE. The suspension was heated for 10 min at 37 °C and was submitted to five freeze–thaw cycles. The liposomes were extruded through 400-nm membranes and through 200-nm membranes. β-OG was then added to reach a 3.4 detergent/lipid ratio (w/w). Proteins were added to the solubilized liposome suspension at the ratio (w/w): lipids/OprM=20. Detergent removal was achieved on addition of Bio-beads at a Bio-bead/detergent ratio of 30 (w/w). The proteoliposomes were concentrated fourfold using an Amicon centrifugal filter (cutoff 100 kDa) and then purified using source Q column (GE Healthcare). The column was extensively washed with 5 M NaCl and 1 N NaOH after the application of each type of liposome. The efficiency of the reconstitution should be systematically controlled by performing ultracentrifugation of the liposomes on a sucrose gradient ( Supplementary Fig. 10 ). Fluorescence assay Fluorescence measurements were conducted at 20 °C using a SAFAS-Xenius spectrofluorimeter. The measurements were performed using the dual-wavelength mode, λ ex =300 nm, λ em =600 nm and λ ex =455 nm, λ em =509 nm. Measurements were performed as triplicates. How to cite this article: Verchère, A. et al . In vitro transport activity of the fully assembled MexAB-OprM efflux pump from Pseudomonas aeruginosa . Nat. Commun . 6:6890 doi: 10.1038/ncomms7890 (2015).